Kindlin-1 regulates mitotic spindle formation by interacting with integrins and Plk-1 Kindlin-1 binds to integrins and regulates integrin activation at cell adhesions. Here we report a new function of Kindlin-1 in regulating spindle assembly. We show that Kindlin-1 localizes to centrosomes, its concentration peaking during G2/M, where it associates with various pericentriolar material proteins, including Polo-like kinase 1. Short interfering RNA-mediated depletion of Kindlin-1 increases formation of abnormal mitotic spindles and decreases cellular survival. This effect is dependent not only on the ability of Kindlin-1 to bind integrins but also on Polo-like kinase 1-mediated Kindlin-1 phosphorylation. We demonstrate that a subcellular pool of phosphorylated Kindlin-1 is located exclusively at centrosomes. Our work identifies a novel cellular role for Kindlin-1 in ensuring mitotic spindle assembly and cellular survival that is controlled by phosphorylation via Polo-like kinase 1. Kindlin-1 (Kin-1) is one of three closely related proteins (Kin-1, -2 and -3) that are present in the human genome. They consist primarily of a four.1, ezrin, radixin and moesin (FERM) domain split by a pleckstrin homology domain. All three kindlins have been shown to bind and regulate integrin activation and also to localize at integrin adhesions [1] , [2] , [3] . Kin-1 is expressed predominantly in epithelial tissues of the skin and intestine, and loss of Kin-1 function in humans results in Kindler Syndrome (KS). Symptoms of KS include skin fragility and blistering [4] , while keratinocytes from KS patients show decreases in substrate adhesion, migration and cell proliferation when compared with keratinocytes from healthy subjects [5] . Genetic deletion of Kin-1 in the mouse leads to skin and intestinal epithelial defects, which are thought to be linked to perturbed integrin activation [6] . Apart from cell-substrate adhesion, integrin activation is also critical for cellular processes such as cell cycle progression [7] , [8] . Disruption of integrin activation leads to defects not only in bipolar spindle assembly but also in their orientation. During interphase, disruption of integrin activation inhibits assembly of microtubules from centrosomes, which subsequently leads to defective bipolar spindles during mitosis. During mitosis, disruption of integrin activation leads to destabilization of astral microtubules, resulting in spindle orientation defects. Little is known of how integrin activation at the cell periphery is transmitted to centrosomes to cause defects in spindle assembly and orientation. Early events critical to setting up bipolar spindles revolve around centrosome duplication, maturation and splitting [9] . The centrosome is the main microtubule organizing centre in animal cells and a number of proteins (including Cdk5rap2, γ-tubulin, Sgo1, hSas, Cep135 and Eg5) and key kinases (such as Polo-like kinases (Plk-1 and Plk-4), Aurora kinase A (Aik-A), Nek-2 and Mst-2) have critical roles in its biology. Centrosome duplication occurs early in S-phase of the cell cycle and is thought to involve Plk-4, hSas and Cep135. Cdk5rap2, Plk-1 and Aik-A then have a central role in centrosome maturation where they help to recruit a number of other proteins, which are collectively known as the pericentriolar material (PCM), to the local vicinity of the centrosome [10] . Once mature, the centrosomes split through the actions of Nek-2, Mst-2 and Eg5, and are then positioned in a bipolar manner, parallel to the cell substrate. The mechanisms by which loss of Kin-1 causes such profound effects in tissues are not fully understood and thus may involve function(s) out-with of cell-substrate adhesion. Interestingly, Kin-1 also localizes to speckles within the nucleus, to the plasma membrane and to the cytosol [4] , [11] , where its function(s) are currently unknown. Here we report on a novel role for Kin-1 at centrosomes in regulating spindle formation during mitosis, which is dependent on both integrin activation and phosphorylation by Plk-1. Using a Kin-1 mutant that is resistant to phosphorylation by Plk-1, we are able to decouple the integrin regulating function of Kin-1 from its function at centrosomes. We propose a novel role for Kin-1 in ensuring proper coordination between the cell cycle and adhesion. Kin-1 regulates spindle assembly via integrin binding Because of their similarity, Kin-1 and -2 likely share at least some redundant roles [11] , [12] ; hence, we studied the cellular role of Kin-1 in MDA-MB-231 breast cancer cells as they express readily detectable levels of Kin-1 and no obvious Kin-2. This was used as the breast cancer cell line of choice as other breast cancer cell lines express both isoforms ( Supplementary Fig. S1a ). As expected, Kin-1 was enriched at integrin adhesions where it colocalized with active focal adhesion kinase (FAK) ( Fig. 1a , white arrowheads). However, not all cells showed robust integrin adhesions, and closer examination revealed these cells to be mitotic. In Fig. 1b (left image), two cells in the same field are shown (one non-mitotic cell, Cell 1, and another undergoing mitosis, Cell 2; further example shown in Supplementary Fig. S1b ); whereas Cell 1 has multiple regions showing Kin-1 enrichment in the adhesion plane ( Fig. 1b ; images, left panels white arrowheads), Cell 2 does not. In Cell 2 (mitotic cell), Kin-1 enrichment was instead observed at the spindle poles in the mitotic plane ( Fig. 1b , images, right panels white arrowheads). Kin-1 localization at other reported locations, such as the plasma membrane and in the cytosol, was similar in mitotic and non-mitotic cells ( Supplementary Fig. S1c ). Talin-1 and vinculin, other prominent adhesion proteins, were not seen prominently localized at spindle poles ( Supplementary Fig. S1d,e ), suggesting that Kin-1 localization at spindle poles is not a general property of all adhesion proteins. 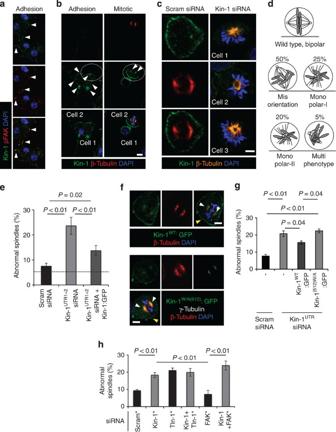Figure 1: The role of Kin-1 in regulating spindle assembly is dependent on integrin binding and activation. (a) Kin-1 colocalizes with activated FAK (tyrosine 397 phosphorylated, pFAK) at focal adhesions, in non-mitotic cells (white arrowheads; scale bar, 8 μm). (b) Kin-1 is enriched at multiple sites along the adhesion plane of Cell 1 (left panels, white arrowheads) and at the spindle poles in Cell 2 in the mitotic plane (right panels, white arrowheads; scale bar, 8 μm). For visualization purposes, the outline of the mitotic cell (Cell 2, dashed white oval) has been shown. (c) siRNA-mediated Kin-1 depletion leads to abnormal spindle formation (Kin-1 siRNA, right column of images, three cells are shown). A non-targeting siRNA (Scram siRNA)-treated cell is shown as control (left panel of images; scale bar, 4 μm). (d) Schematic of a bipolar wild-type spindle and the breakdown of the four abnormal spindle phenotypes seen upon Kin-1 depletion (Misorientation, Monopolar-I, Monopolar-II and Multi-phenotype). The grey line represents the substrate the cells are adhered to, and misorientated spindles were defined as spindles that were not parallel to the substrate. (e) Quantification of the incidence of abnormal spindles in Scram siRNA, Kin-1UTR1+2siRNA and Kin-1UTR1+2siRNA plus Kin-1:GFP-expressing cells (n=8, ±s.e.m., ≥250 spindles scored for each condition). The dashed black line corresponds to the average percentage of abnormal spindle incidence in untreated control cells (5.3±1.9,n=3, ±s.e.m, ≥250 spindles scored). (f) Kin-1:GFP and Kin-1W/A(612):GFP both localize to the spindle poles of mitotic cells (white arrowheads) as well as to the plasma membrane (yellow arrowhead; scale bar, 8 μm). (g) Quantification of the incidence of abnormal spindles in Scram siRNA, Kin-1UTR1+2siRNA, Kin-1UTR1+2siRNA plus Kin-1:GFP and Kin-1UTR1+2siRNA plus Kin-1W/A(612):GFP-expressing cells (n=4, ±s.e.m., ≥250 spindles scored for each condition). (h) Kin-1 and talin-1 siRNA treatment both resulted in a similar increase in mutant spindles formation, whereas FAK siRNA had no effect. There was no co-operative increase in mutant spindles when both Kin-1 and talin were depleted (n=4, ±s.e.m., ≥250 spindles scored for each condition). Student’st-tests were performed where indicated. Figure 1: The role of Kin-1 in regulating spindle assembly is dependent on integrin binding and activation. ( a ) Kin-1 colocalizes with activated FAK (tyrosine 397 phosphorylated, pFAK) at focal adhesions, in non-mitotic cells (white arrowheads; scale bar, 8 μm). ( b ) Kin-1 is enriched at multiple sites along the adhesion plane of Cell 1 (left panels, white arrowheads) and at the spindle poles in Cell 2 in the mitotic plane (right panels, white arrowheads; scale bar, 8 μm). For visualization purposes, the outline of the mitotic cell (Cell 2, dashed white oval) has been shown. ( c ) siRNA-mediated Kin-1 depletion leads to abnormal spindle formation (Kin-1 siRNA, right column of images, three cells are shown). A non-targeting siRNA (Scram siRNA)-treated cell is shown as control (left panel of images; scale bar, 4 μm). ( d ) Schematic of a bipolar wild-type spindle and the breakdown of the four abnormal spindle phenotypes seen upon Kin-1 depletion (Misorientation, Monopolar-I, Monopolar-II and Multi-phenotype). The grey line represents the substrate the cells are adhered to, and misorientated spindles were defined as spindles that were not parallel to the substrate. ( e ) Quantification of the incidence of abnormal spindles in Scram siRNA, Kin-1 UTR1+2 siRNA and Kin-1 UTR1+2 siRNA plus Kin-1:GFP-expressing cells ( n =8, ±s.e.m., ≥250 spindles scored for each condition). The dashed black line corresponds to the average percentage of abnormal spindle incidence in untreated control cells (5.3±1.9, n =3, ±s.e.m, ≥250 spindles scored). ( f ) Kin-1:GFP and Kin-1 W/A(612) :GFP both localize to the spindle poles of mitotic cells (white arrowheads) as well as to the plasma membrane (yellow arrowhead; scale bar, 8 μm). ( g ) Quantification of the incidence of abnormal spindles in Scram siRNA, Kin-1 UTR1+2 siRNA, Kin-1 UTR1+2 siRNA plus Kin-1:GFP and Kin-1 UTR1+2 siRNA plus Kin-1 W/A(612) :GFP-expressing cells ( n =4, ±s.e.m., ≥250 spindles scored for each condition). ( h ) Kin-1 and talin-1 siRNA treatment both resulted in a similar increase in mutant spindles formation, whereas FAK siRNA had no effect. There was no co-operative increase in mutant spindles when both Kin-1 and talin were depleted ( n =4, ±s.e.m., ≥250 spindles scored for each condition). Student’s t -tests were performed where indicated. Full size image Depletion of integrins has already been shown to lead to defects during mitosis and, in particular, in forming normal bipolar spindles [7] . As Kin-1 is a critical regulator of integrin activation, we depleted Kin-1 in synchronized cells to determine whether this would also lead to defects in mitotic spindles. Fluorescence-activated cell sorting demonstrated that following a thymidine block, cells were effectively trapped in G1/S, and that 6 h after release (by removal of thymidine) around 75% of the cells were in G2/M when mitotic spindles were analysed ( Supplementary Fig. S1f ). Short interfering RNA (siRNA)-induced depletion of Kin-1 ( Supplementary Fig. S1g ) led to an increase in abnormal mitotic spindles and in particular misorientated and monopolar spindles ( Fig. 1c , and schematically depicted in Fig. 1d ). Misorientated spindles accounted for 50% of the abnormal phenotype, while monopolar spindles accounted for 45%. The monopolar spindles can be further subdivided into spindles that had one or two identifiable centrosomes. The third type of mutant spindles (5%) consisted of spindles that either straddled the two dominant types of spindles or were multipolar (~1% of mutant spindles). We also examined the effects of individual Kin-1 siRNA sequences, which showed the same spindle defects, and there was a correlation between degree of knockdown of Kin-1 by individual sequences and the proportion of mutant spindles ( Supplementary Fig. S1g ). To control for off-target effects of the siRNA, we expressed an siRNA-resistant Kin-1 fused to GFP (Kin1:GFP) at the same time as siRNA directed to the untranslated region of endogenous Kin-1 mRNA to deplete endogenous Kin-1. Quantification of the mutant spindle phenotype induced by siRNA depletion of Kin-1 was then determined. Specifically, around 93–95% of cells treated with scrambled siRNA had bipolar, apparently wild-type spindles, with ~5–7% having abnormal spindles ( Fig. 1e ). However, around 25% of cells depleted of Kin-1 had abnormal spindles. Re-expression of Kin-1:GFP resulted in partial rescue of the abnormal spindle phenotype seen after knockdown of endogenous Kin-1; the partial rescue of the spindle phenotype is likely due to the lower level of expression of exogenous tagged Kin-1:GFP achieved, compared with endogenous levels of Kin-1 in scrambled siRNA control cells ( Supplementary Fig. S1h ). We next asked whether the function of Kin-1 at adhesions is important for normal spindle assembly. Tryptophan (W) 612 within Kin-1 is critical for integrin binding and its mutation to alanine (A) (Kin-1 612(W/A) ) renders it unable to bind integrins [1] . As with endogenous Kin-1, expression of Kin-1:GFP (in Kin-1-depleted cells) was able to localize to spindle poles ( Fig. 1f , top panel images, white arrowheads) in mitotic cells and also to the plasma membrane ( Fig. 1f , yellow arrowhead). Although Kin-1 612(W/A) fused to GFP (Kin-1 612(W/A) :GFP) was able to associate with centrosomes ( Fig. 1f , bottom panel images), it was unable to rescue the increased abnormal spindle formation due to Kin-1 depletion, as compared with the expression of wild-type Kin-1:GFP ( Fig. 1g ). To confirm a requirement for integrin activation in the abnormal spindle phenotype, we treated cells with the Arg-Gly-Asp (RGD) integrin-binding peptide, which inhibits full integrin-mediated signalling [13] . Treatment with RGD peptide resulted in a dose-dependent increase in the number of mutant spindles ( Supplementary Fig. S1i ). No further increase in mutant spindles was seen when Kin-1 knockdown cells were treated with RGD peptide. siRNA-mediated deletion of talin, another FERM domain protein that is required for integrin activation, also induced spindle defects, and this was not further increased when Kin-1 expression was knocked down ( Fig. 1h and Supplementary Fig. S1j ). In contrast, siRNA-mediated depletion of FAK, which is activated downstream of integrin engagement, had no effect on spindle formation. Taken together, these data imply that the effects of Kin-1 on spindle formation are linked to its ability to bind and activate integrins at the cell membrane. Kin-1 is a PCM protein We next examined Kin-1 localization in cells more precisely to help determine the role of Kin-1 at centrosomes. This was done in two ways; first, by determining when in the cell cycle Kin-1 localization at centrosomes was maximal and, second, which centrosomal proteins Kin-1 colocalized with. In cells arrested in G1/S ( Supplementary Fig. S1f ), there was no detectable Kin-1 associated with centrosomes ( Fig. 2a , 0 h), whereas mitotic cells (6 h) always displayed Kin-1 localization at centrosomes ( Fig. 2a ; white arrowheads indicate Kin-1 localization at centrosomes and orange arrowheads indicate no detectable Kin-1 at centrosomes). This increase in the number of cells displaying localization of Kin-1 at centrosomes as cells approach mitosis, correlates with the timing of centrosome maturation. Throughout the cell cycle, Kin-1 was always present at the plasma membrane (red arrowheads) and in the cytosol. 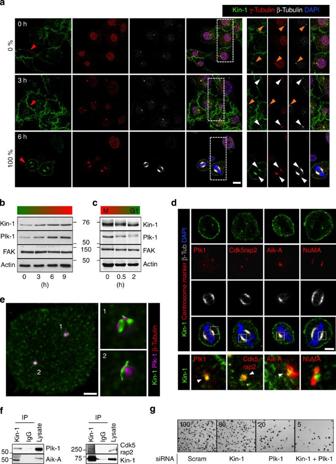Figure 2: Kin-1 is a PCM protein. (a) Kin-1 localization at centrosomes is absent in cells at G1/S (orange arrowheads) but localizes there as cells enter G2/M (white arrowheads; scale bar, 15 μm). During mitosis, all centrosomes show Kin-1 localization. γ-tubulin is used to mark centrosomes and red arrow heads indicate plasma membrane localization of Kin-1. (b) Western analysis for Kin-1 from lysate of MDA-MB-231 cells arrested at G1/S (0 h) and at time points after release. Kin-1 and Plk-1 levels are higher at G2/M (6 h after release from G1/S arrest) than at G1/S. (c) As cells exit mitosis, Kin-1 and Plk-1 levels are reduced. (d) Costaining of Kin-1 with prominent centrosome markers Plk-1, Cdk5rap-2, Aik-A and NuMA (white arrowheads). Boxed centrosomes in the merged images are enlarged in the bottom panels. Kin-1 (green) and centrosome marker (red; scale bar, 8 μm). (e) Volume rendered three-dimensional presentation of Kin-1 (green) and Plk-1 (magenta) colocalization at centrosomes in a mitotic cell (left; scale bar, 2 μm). Surface rendering of the centrosome immunofluorescence is shown in the right images. (f) Kin-1-specific antibodies were able to coimmunoprecipitate (IP) Plk-1, Aik-A and Cdk5rap2. (g) siRNA-mediated depletion of Kin-1 and Plk-1 results in decreased cell survival as assayed by clonogenic assays. Simultaneous depletion of Kin-1 and Plk-1 results in a further decrease in cell survival compared with depletion of either alone. The percentage of colonies relative to colonies returned with non-targeting siRNA-treated cells is indicated top left. Figure 2: Kin-1 is a PCM protein. ( a ) Kin-1 localization at centrosomes is absent in cells at G1/S (orange arrowheads) but localizes there as cells enter G2/M (white arrowheads; scale bar, 15 μm). During mitosis, all centrosomes show Kin-1 localization. γ-tubulin is used to mark centrosomes and red arrow heads indicate plasma membrane localization of Kin-1. ( b ) Western analysis for Kin-1 from lysate of MDA-MB-231 cells arrested at G1/S (0 h) and at time points after release. Kin-1 and Plk-1 levels are higher at G2/M (6 h after release from G1/S arrest) than at G1/S. ( c ) As cells exit mitosis, Kin-1 and Plk-1 levels are reduced. ( d ) Costaining of Kin-1 with prominent centrosome markers Plk-1, Cdk5rap-2, Aik-A and NuMA (white arrowheads). Boxed centrosomes in the merged images are enlarged in the bottom panels. Kin-1 (green) and centrosome marker (red; scale bar, 8 μm). ( e ) Volume rendered three-dimensional presentation of Kin-1 (green) and Plk-1 (magenta) colocalization at centrosomes in a mitotic cell (left; scale bar, 2 μm). Surface rendering of the centrosome immunofluorescence is shown in the right images. ( f ) Kin-1-specific antibodies were able to coimmunoprecipitate (IP) Plk-1, Aik-A and Cdk5rap2. ( g ) siRNA-mediated depletion of Kin-1 and Plk-1 results in decreased cell survival as assayed by clonogenic assays. Simultaneous depletion of Kin-1 and Plk-1 results in a further decrease in cell survival compared with depletion of either alone. The percentage of colonies relative to colonies returned with non-targeting siRNA-treated cells is indicated top left. Full size image Many proteins are involved in the regulation of centrosome maturation [10] and, importantly, disruption of these proteins leads to defects in spindle formation similar to the defects seen with Kin-1 depletion [14] , [15] , [16] . Such proteins are collectively known as PCM proteins and include Plk-1, Cdk5rap2 and Aik-A. Further, most PCM proteins are subject to cell-cycle-dependent regulation of their activity and expression. We found that Kin-1 levels increased as cells progressed from G1/S (0 h) to G2/M (6 h), which mirrored the changes in Plk-1 and Aik-A expression ( Fig. 2b ). In contrast, there was no change in total FAK, another FERM domain-containing adhesion protein ( Fig. 2b ). Once mitosis is complete, most PCM proteins are subject to protein degradation, which leads to loss of expression. To test whether this was also true for Kin-1, cells were arrested in prometaphase using nocodazole and released to allow completion of mitosis. As with Plk-1 and Aik-A, Kin-1 levels were also reduced as cells exited mitosis ( Fig. 2c ). Thus, Kin-1 levels are regulated in a similar manner to other established and critical cell cycle regulators. The roles of many PCM proteins at centrosomes have been extensively characterized [10] and we next carried out colocalization and coimmunoprecipitation studies with prominent PCM proteins. Critical centrosomal/PCM proteins, Plk-1, Aik-A, NuMA (ref. 16 ) and Cdk5rap2, all show some degree of colocalization with Kin-1 ( Fig. 2d ). A closer examination of the boxed centrosomes ( Fig. 2d , merged images, dashed white boxes) suggested that Kin-1 colocalized most tightly with Plk-1 and Cdk5rap2 ( Fig. 2d , merged images bottom panel). High-resolution microscopy followed by deconvolution with volume and surface rendering was applied to more precisely map and illustrate the localization of Kin-1 at centrosomes ( Fig. 2e and Supplementary Fig. S2a–c ). Kin-1 shares significant areas of colocalization with Plk-1 and Cdk5rap2 at centrosomes, as well as localizing to unique areas out with of either. Immunoprecipitation using a Kin-1-specific antibody was able to coimmunoprecipitate Plk-1, Aik-A and Cdk5rap2 ( Fig. 2f ). Conversely, immunoprecipitation using a Plk-1-specific antibody was able to coimmunoprecipitate Kin-1 ( Supplementary Fig. S2d ). The interaction with Plk-1 was direct as recombinant Plk-1 was preferentially pulled down by glutathione S -transferase (GST) fused to Kin-1 (GST:Kin-1) over GST alone ( Supplementary Fig. S2e ). Further, this binding was only partially sensitive to the Plk-1 Polo-box-domain-targeting drug thymoquinone [17] ( Supplementary Fig. S2f ), suggesting that other parts of the protein outside of the Polo-box domain are involved in the interaction. Thus, Kin-1 both colocalized and associated with a number of critical PCM proteins (Plk-1, Cdk5rap2 and Aik-A). Its protein levels were regulated as other PCM proteins during the cell cycle and, as with many other PCM proteins, Kin-1 depletion led to abnormal spindle formation. The likely consequence of abnormal spindles is eventual cell death, which is seen following depletion of other PCM proteins, including Plk-1, Aik-A and Cdk5rap2. Therefore, clonogenic assays were carried out to determine the consequence of Kin-1 depletion on cell survival ( Fig. 2g ). siRNA-mediated depletion of Kin-1 led to a significant decrease in cell survival (20%) compared with scrambled siRNA control. Although siRNA-mediated depletion of Plk-1 led to a significant decrease in cell survival (80% compared with control), depletion of both Kin-1 and Plk-1 simultaneously resulted in an enhanced effect with up to a 95% decrease in cell survival (quantified in Supplementary Fig. S2g ). Taken together, these data suggest that Kin-1 itself is a PCM protein and, as such, may have a critical role in mitotic spindle formation. Kin-1 localization to centrosomes is Plk-1 dependent The localization of PCM proteins to centrosomes is complex and requires the interplay of multiple proteins and pathways. Plk-1, Aik-A and Cdk5rap2 represent critical components that regulate centrosome maturation by influencing the localization of many other PCM proteins. Thus, we tested the dependence of Kin-1 localization to centrosomes on these three components by the use of siRNA-induced protein depletion ( Fig. 3a ). Cells treated with non-targeting siRNA oligos (Scram) formed normal, bipolar spindles and Kin-1 colocalized with γ-tubulin at centrosomes ( Fig. 3a , left panels, white arrowheads). In cells depleted of Aik-A and Cdk5rap2 ( Supplementary Fig. S3a ), Kin-1 still localized to centrosomes, even in cells with abnormal spindles ( Fig. 3a , white arrowheads). However, in cells depleted of Plk-1, Kin-1 localization was greatly reduced or lost at centrosomes ( Fig. 3a ). Thus, Plk-1 is required for localization of Kin-1 to centrosomes. Depletion of Kin-1 had little to no effect on the ability of Plk-1 or Cdk5rap2 to localize to spindle poles ( Supplementary Fig. S3b,c ). 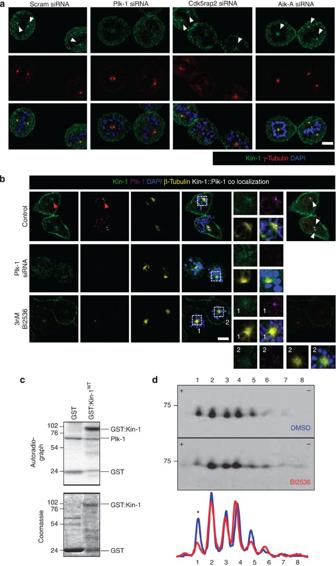Figure 3: Kin-1 localization at centrosomes and its phosphorylation status depend on Plk-1. (a) siRNA-induced depletion of Plk-1, but not Cdk5rap2 or Aik-A, resulted in loss of Kin-1 (green) staining from centrosomes. Centrosomes are labelled with anit-γ-tubulin (red). White arrowheads indicate colocalization with Kin-1 (scale bar, 8 μm). (b) siRNA-induced depletion of Plk-1 or treatment of cells with 3 nM BI2536 results in reduced localization of Kin-1 to centrosomes/spindle poles (scale bar, 15 μm). The ‘Colocalization Threshold’ function in FIJI image software was used to determine the extent of colocalization between Kin-1 and Plk-1 (far right panels). (c) Recombinant Plk-1 is able to phosphorylate GST fused to Kin-1 (GST:Kin-1). (d) Two-dimensional SDS–PAGE analysis of Kin-1 reveals up to eight different Kin-1 isoforms (spots 1–8, top blot). Treatment with 15 nM BI2536 for 8 h resulted in the reduction of spot 1 (bottom blot) compared with control (n=2, representative blots shown). Densitometry of the spots was determined using the ‘Plot profile’ feature in FIJI image software and their values plotted and overlaid to more clearly represent the change in the intensity of spot 1 (*) upon BI2536 treatment. Figure 3: Kin-1 localization at centrosomes and its phosphorylation status depend on Plk-1. ( a ) siRNA-induced depletion of Plk-1, but not Cdk5rap2 or Aik-A, resulted in loss of Kin-1 (green) staining from centrosomes. Centrosomes are labelled with anit-γ-tubulin (red). White arrowheads indicate colocalization with Kin-1 (scale bar, 8 μm). ( b ) siRNA-induced depletion of Plk-1 or treatment of cells with 3 nM BI2536 results in reduced localization of Kin-1 to centrosomes/spindle poles (scale bar, 15 μm). The ‘Colocalization Threshold’ function in FIJI image software was used to determine the extent of colocalization between Kin-1 and Plk-1 (far right panels). ( c ) Recombinant Plk-1 is able to phosphorylate GST fused to Kin-1 (GST:Kin-1). ( d ) Two-dimensional SDS–PAGE analysis of Kin-1 reveals up to eight different Kin-1 isoforms (spots 1–8, top blot). Treatment with 15 nM BI2536 for 8 h resulted in the reduction of spot 1 (bottom blot) compared with control ( n =2, representative blots shown). Densitometry of the spots was determined using the ‘Plot profile’ feature in FIJI image software and their values plotted and overlaid to more clearly represent the change in the intensity of spot 1 (*) upon BI2536 treatment. Full size image BI2536 is a highly specific inhibitor that targets the kinase activity of Plk-1 (ref. 18 ). To determine whether the kinase activity or the physical interaction between Plk-1 and Kin-1 is critical for Kin-1 localization to centrosomes, mitotic cells depleted of Plk-1 and cells treated with BI2536 were costained with Kin-1, Plk-1 and β-tubulin ( Fig. 3b ). Dose dependence of BI2536 on cell proliferation and its ability to induce abnormal spindles was first determined ( Supplementary Fig. S3d,e ). Control cells formed bipolar spindles where Kin-1 and Plk-1 colocalized strongly. ( Fig. 3b , top panel). The areas where Kin-1 and Plk-1 colocalized within cells were confirmed objectively using FIGI software (‘colocalization threshold’ function) and are indicated by white arrowheads. Cells depleted of Plk-1 resulted in abnormal, largely monopolar spindles ( Fig. 3b , middle panel). In these cells, Kin-1 was not obviously concentrated at the spindle poles (where centrosomes normally reside), appearing instead to be more diffusely located in the cytoplasm ( Fig. 3b , middle panel). As with Plk-1 knockdown, BI2536 treatment led to the formation of abnormal spindles. In some cells, Plk-1 could be seen diffusely around the spindle poles, and in these cases Kin-1 staining was also diffuse around the spindle poles ( Fig. 3b , lower panel, inset 1). In the cells where Plk-1 was still clearly visible at the spindle poles, Kin-1 was able to colocalize with Plk-1; however, the level of colocalization was greatly reduced compared with controls ( Fig. 3b , bottom panel, inset 2). Precise Kin-1 overlap with Plk-1 localization was not as strong as in control situations when objective colocalization analysis was performed ( Fig. 3b , far right images). Thus, as Plk-1 levels and activity are both required for proper centrosomes maturation [19] ; without them, the precise localization of Kin-1 to the vicinity of centrosomes is greatly impaired. As Plk-1 is a critical cell cycle kinase, we next asked whether Kin-1 was a substrate of Plk-1. Recombinant Plk-1 was able to directly phosphorylate GST fused to Kin-1 in vitro ( Fig. 3c ). Using two-dimensional SDS–polyacrylamide gel electrophoresis we determined the phosphorylation status of Kin-1 in cells and whether it was sensitive to Plk-1 activity ( Fig. 3d ). We found Kin-1 existed in at least eight different post-translationally modified isoforms (presumably representative of different phosphorylation states) in cells ( Fig. 3d , top blot and blue spot intensity profile). To inhibit Plk-1 activity, we treated cells with BI2536 for 8 h, which revealed that one form (isoform 1) was sensitive to BI2536 treatment ( Fig. 3d , bottom blot and red spot intensity profile). Thus, Plk-1 regulates the localization and the phosphorylation status of Kin-1 in cells and is able to phosphorylate Kin-1 directly in vitro . Kin-1 phosphorylation is required for spindle formation Sequence analysis of Kin-1 suggested two strong potential Plk-1 phosphorylation consensus sites on Kin-1 centred around threonine (T) 8 and 30 ( Supplementary Fig. S4a ) [20] . GST fusion proteins consisting of the first 45 amino acids of wild type (GST:45 WT ) and a non-phosphorylatable Kin-1 isoform, where the T residues were mutated to alanine (A) residues (GST:45 (8+30)T/A ), were subject to in vitro kinase assays. GST:45 (8+30)T/A showed greatly reduced phosphorylation compared to GST:45 WT ( Supplementary Fig. S4b ). We next attempted to raise antibodies against Kin-1 phosphorylated at T8 and T30. Because of low antigenicity of the T8 epitope, we were only able to raise an antibody against the phosphorylated T30 epitope (anti-pKin-1 T30 ). The anti-pKin-1 T30 antibody was able to detect endogenous phosphorylated Kin-1 upon western analysis and further increasing doses of BI2536 led to a decrease in T30-phosphorylated Kin-1 (pKin-1 T30 ) in cells ( Fig. 4a ). Exogenous expression of Kin-1 WT :GFP and Kin-1 (8+30)T/A :GFP was used as a further control to validate the specificity of the antibody: anti-pKin-1 T30 , and was able to recognize endogenous Kin-1 and the wild-type Kin-1 protein but not the mutant form of Kin-1 ( Fig. 4b ). Finally, mitotic and 90-min post-mitotic cell lysates were probed using anti-pKin-1 T30 , which showed that Kin-1 phosphorylation was reduced following release from mitosis ( Fig. 4c ). As expected, levels of activated Plk-1 (Plk-1 phosphorylated on T210, pPlk1) were also greatly reduced in the post-mitotic cell lysate. These data show that Kin-1 is subject to phosphorylation by Plk-1 both in vitro and in cells at T30. 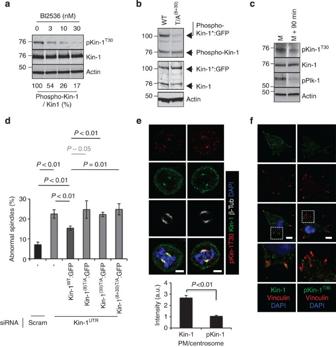Figure 4: Phosphorylation of Kin-1 by Plk-1 is required for the regulation of mitotic spindles. (a) Western analysis using an antibody raised against phosphorylated T30 of Kin-1 (anti-pKin-1T30) showed loss of signal from cell lysate of cells treated with BI2536. Kin-1 and actin are shown as loading controls, and the relative loss of signal (with respect to Kin-1) is shown below. (b) Exogenous expression of Kin-1(8+30)T/A:GFP is not recognized by anti-phospho-Kin-1, whereas endogenous Kin-1 and Kin-1WT:GFP are. (c) Western analysis showed a decrease in Kin-1 phosphorylation at T30 in 90 min post mitotic (M+90) cell lysate compared with mitotic (M) cell lysate. (d) Quantification of the incidence of abnormal spindles in Scram siRNA, Kin-1UTR1+2siRNA and Kin-1UTR1+2siRNA plus expression of wild-type Kin-1 fused to GFP (Kin-1WT:GFP) or mutant Kin-1 isoforms as indicated (n=4, ±s.e.m., ≥250 spindles scored for each condition). (e) Immunostaining of mitotic cells showed that pKin-1T30was present at centrosomes but not at the plasma membrane. In contrast, total Kin-1 was present at both centrosomes and the plasma membrane (scale bar, 4 μm). Quantification of the ratio of staining intensity at the plasma membrane and the centrosome, of total Kin-1 and pKin-1T30, is shown below the panel of two representative cells (n=2, ±s.e.m.). (f) Immunostaining of adhesions with anti-pKin-1T30and anti-vinculin showed that pKin-1T30is absent from adhesions (scale bar, 8 μm). Student’st-tests were performed where indicated. Figure 4: Phosphorylation of Kin-1 by Plk-1 is required for the regulation of mitotic spindles. ( a ) Western analysis using an antibody raised against phosphorylated T30 of Kin-1 (anti-pKin-1 T30 ) showed loss of signal from cell lysate of cells treated with BI2536. Kin-1 and actin are shown as loading controls, and the relative loss of signal (with respect to Kin-1) is shown below. ( b ) Exogenous expression of Kin-1 (8+30)T/A :GFP is not recognized by anti-phospho-Kin-1, whereas endogenous Kin-1 and Kin-1 WT :GFP are. ( c ) Western analysis showed a decrease in Kin-1 phosphorylation at T30 in 90 min post mitotic (M+90) cell lysate compared with mitotic (M) cell lysate. ( d ) Quantification of the incidence of abnormal spindles in Scram siRNA, Kin-1 UTR1+2 siRNA and Kin-1 UTR1+2 siRNA plus expression of wild-type Kin-1 fused to GFP (Kin-1 WT :GFP) or mutant Kin-1 isoforms as indicated ( n =4, ±s.e.m., ≥250 spindles scored for each condition). ( e ) Immunostaining of mitotic cells showed that pKin-1 T30 was present at centrosomes but not at the plasma membrane. In contrast, total Kin-1 was present at both centrosomes and the plasma membrane (scale bar, 4 μm). Quantification of the ratio of staining intensity at the plasma membrane and the centrosome, of total Kin-1 and pKin-1 T30 , is shown below the panel of two representative cells ( n =2, ±s.e.m.). ( f ) Immunostaining of adhesions with anti-pKin-1 T30 and anti-vinculin showed that pKin-1 T30 is absent from adhesions (scale bar, 8 μm). Student’s t -tests were performed where indicated. Full size image To test the biological significance of Kin-1 phosphorylation by Plk-1, we asked whether expression of Kin-1 (8+30)T/A :GFP was able to rescue the abnormal spindle phenotype induced by the depletion of endogenous Kin-1. Expression of Kin-1 (8+30)T/A :GFP failed to rescue the phenotype and nor did expression of the individual mutants ( Fig. 4d ). Expression of activated β1-integrin, as measured using an antibody (9EG7) that recognizes the activated β1-integrin associated epitope [6] , [21] , was similar in both Kin-1 (8+30)T/A :GFP and Kin-1 WT :GFP expressing cells that were also depleted for endogenous Kin-1 ( Supplementary Fig. S4c ). In contrast, Kin-1-depleted cells expressing the non-integrin binding mutant Kin-1 (612)W/A :GFP showed significantly reduced levels of β1-integrin activation ( Supplementary Fig. S4c ). Further, both Kin-1 (8+30)T/A :GFP and Kin-1 WT :GFP were able to colocalize with the prominent adhesion markers paxillin and phospho (Y-416)-Src at adhesions ( Supplementary Fig. S4d ). Thus, although the spindle-associated function of Kin-1 is perturbed in the Kin-1 (8+30)T/A :GFP mutant, its integrin-associated function remains intact. Finally, we found that pKin-1 T30 preferentially localized to centrosomes with only limited staining seen at the plasma membrane ( Fig. 4e ). Whereas total Kin-1 costained with the adhesion marker vinculin, pKin-1 T30 was not detectable at vinculin adhesion sites ( Fig. 4f ). Taken together, these data demonstrate that Kin-1 is a substrate for Plk-1 and that phosphorylated Kin-1 at the centrosome is critical for the ability of Kin-1 to regulate normal spindle assembly. Previous to this work, Kin-1 loss was known to induce keratinocyte adhesion, spreading and migration defects that were attributed to impaired integrin activation [22] . Ubiquitous Kin-1 loss in the mouse results in perinatal lethality due to severe intestinal dysfunction, with the detachment of colonic epithelium as a result of impaired integrin activation [6] . Here we have identified a role for Kin-1 in the regulation of the mitotic spindle. Although the data presented here focused on MDA-MB-231 breast cancer cells where Kin-1 expression is relatively high, we also found that Kin-1 localized at centrosomes in normal mouse keratinocytes ( Supplementary Fig. S4e ) and colocalized with Plk-1 in MCF-10A breast epithelial cells ( Supplementary Fig. S4f ) and Hela cells ( Supplementary Fig. S4g ). Depletion of Kin-1 in MCF-10A cells also caused a significant increase in abnormal spindles ( Supplementary Fig. S4h ). Interestingly, these cells express both Kin-1 and Kin-2, indicating that Kin-2 cannot compensate for the loss of Kin-1. Further, studies are required to determine whether Kin-2 does have a role at centrosomes. However, centrosomal localization and regulation of spindle formation is a function of Kin-1 in multiple cell types. Orientation of the spindle is regulated by β1-integrin via a mechanism involving accumulation of phosphatidylinositol-3,4,5-triphosphate (PtdIns(3,4,5)P3) at the mid-cortex, which in turn regulates dynein/dynactin contractile forces that control spindle orientation [23] . Integrins are also involved in the regulation of microtubules and spindle assembly, with disruption of integrin signalling causing formation of misorientated spindles, although the mechanisms involved are not yet known [7] . The phenotype of abnormal spindles induced by Kin-1 depletion parallels the phenotypes observed by integrin disruption and disruption of PCM members, such as Plk-1, Cdk5rap2 and Aik-A. Whereas integrin disruption leads primarily to spindle orientation defects, disruption of PCM proteins leads not only to spindle orientation defects but also to defects in centrosome maturation, duplication, division and spindle stability. The phenotype we observed upon depletion of Kin-1 encompasses not only spindle orientation defects but also defects in centrosome division and/or separation. The later phenotypes suggest an additional role for Kin-1 than simply transducing integrin signalling from the cortex. This is supported by our observation that Kin-1 is phosphorylated by Plk1 at centrosomes (and not at adhesions) and that this phosphorylation is required for normal spindle formation. Further, expression of the Plk-1 phosphorylation-resistant mutant of Kin-1 (Kin-1 (8+30)T/A) ) in Kin-1-depleted cells is still able to activate integrins to the same extent as wild-type Kin-1. Therefore, Kin-1 controls spindle formation via regulation of integrin activation and also through its phosphorylation at centrosomes. Although the specific role of Kin-1 at centrosomes is still unclear, it may be similar to the role it serves at integrin adhesions, where it functions as an adaptor/scaffold protein to help initiate integrin-linked adhesion complexes. A critical process in centrosome maturation is in the recruitment and turnover of PCM proteins and although Kin-1 is not required for the recruitment of critical PCM components (Plk-1, Cdk5rap-2 or Aik-A), it may be required for the recruitment of other proteins that are required for normal mitosis. We propose that there is ‘communication’ between integrin adhesions and the PCM and that Kin-1 may act as a ‘status sensing’ molecule to co-ordinate adhesion/de-adhesion with proper spindle assembly and mitosis. Cell culture and transfection MDA-MB-231 (American Type Culture Collection) cells were cultured using DMEM (Gibco) supplemented with 10% fetal calf serum (Gibco) and glutamine under standard conditions of 37 °C and 5% CO 2 . The MDA-MB-231 Amaxa transfection protocol was used to transfect cells with siRNA (100 nM) and/or plasmid DNA (0.5 μg). All plasmids used were based on pEGFP-N1 backbone (Clontech Laboratories Inc.). For transfections plus cell cycle treatments, transfections were carried out 8 h before start of the double thymidine arrest protocol. All siRNA oligos were purchased from Dharmacon RNAi Technologies (Kin-1 siRNA Pool, E-004511-14-0005 (5′-UCUUACGAUUUAAAUAUUA-3′, 5′- UCCUUAUCUACAGUUGAUU-3′, 5′-CUAUUAUUUUAGAACCUAG-3′, 5′-CCAUGACCCCUAUAUAUGA-3′); Kin-1 siRNA UTR1, A004511-14-0005 (5′-UCCUUAUCUACAGUUGAUU-3′); Kin-1 siRNA UTR2, A004511-15-0005 (5′-CUAUUAUUUUAGAACCUAG-3′); and non-targeting siRNA, D-001910-0105; Talin-1 siRNA pool, L-012949-00-0005 (5′-GAAGAUGGUUGGCGGCAUU-3′, 5′-GUAGAGGACCUGACAACAA-3′, 5′-UCAAUCAGCUCAUCACUAU-3′, 5′-GAGAUGAGGAGUCUACUAU-3′); FAK siRNA pool, L003164-00-0005 (5′-GCGAUUAUAUGUUAGAGAU-3′, 5′-GGGCAUCAUUCAGAAGAUA-3′, 5′-UAGUACAGCUCUUGCAUAU-3′, 5′-GGACAUUAUUGGCCACUGU-3′); and Cdk5rap2 siRNA pool, EU-019154-00-0002 (5′-GCCAUAAUUACAGUUUUGU-3′, 5′-CGGUCAUUAGGAAAUAUGU-3′, 5′-CCAUGGCAUUAAAAUCAAA-3′ and 5′-GUGUGGUUCCUAUUUAUUG-3′)). For Kin-1 siRNA treatment, the pool was used throughout unless otherwise stated. The double thymidine block protocol was used to arrest cells at G1/S. Cells were treated with two successive incubations of 2 mM thymidine (for 17 h and 14 h) 8 h apart. Plk-1-specific inhibitor (BI2536; 1 nM) or RGD peptide (Enzo, BML-P700-0005) was added to cells upon release of cells from the second thymidine incubation. The extent of cell cycle arrest was verified by fixing cells in 70% ethanol followed by nuclear staining using propidium iodide and flow cytometric analysis. For arrest of cells in prometaphase, cells were treated with 32 nM nocodazole for 16 h. Western analysis and immunofluorescence Cells for western analysis were lysed using RIPA buffer (25 mM Tris, 150 mM NaCl (TBS), 1% DOC, 0.1% SDS, pH 7.6) plus protease and phosphatase inhibitors (aprotinin, leupeptin, PMSF, benzamidine and sodium orthovanadate). Proteins were separated according to size using SDS–PAGE, transferred onto nitrocellulose membrane and blocked for 1 h in TBS+0.05% Tween-20 (TBST)+5% BSA. Membranes were incubated for 16 h at 4 °C and for 45 min at room temperature for primary and secondary antibodies, respectively. All washes and antibody incubations were carried out in TBST and TBST+5% BSA, respectively. For immumofluorescence analysis, cells were grown on glass coverslips, washed once in TBS, and fixed and permeabilized for 10 min at room temperature in Fix buffer (100 mM PIPES, 3.7% paraformaldehyde, 0.2% Triton X-100, 1 mM MgCl 2 and 10 mM EGTA, pH 7.4). Coverslips were washed twice in wash buffer (TBS plus 0.1% Triton X-100) and incubated with the primary antibody for 16 h at 4 °C in wash buffer+2% BSA. Secondary antibody incubations were carried out for 1 h at room temperature in wash buffer+2% BSA. All washes were carried out with wash buffer. Images were captured using an FV-1000 Olympus confocal microscope using a × 60 objective. For volume (and surface) rendering, cells were immunostained and imaged on a Leica SP5 SMD microscope. Data sets were acquired at Nyquist sampling rates in both the lateral and axial dimensions before deconvolution using theoretical point spread functions using Huygens software (Scientific Volume Imaging). Deconvolved data sets were analysed in three dimensions using Imaris (Bitplane). Antibodies used: anti-Kin-1 (Stratech, H00055612-B01P (1:3,000 for western blotting (WB) and 1:300 for immunofluorescence (IF)) and Abcam, ab68041); anti-phospho (T30) Kin-1 (generated through Eurogentec (1:500 for WB and 1:75 for IF)); anti-Plk-1 (Cell Signaling Technology, 4513); anti-Actin (Sigma, A3853 (1:4,000 for WB)); anti-FAK (Cell Signaling Technology, 3285); anti-phospho-FAK 397 (Biosource, 44-625G); anti-Aik-A (Cell Signaling Technology, 4718); anti-NuMA (Cell Signaling Technology, 8967); anti-CDK5RAP2 (Millipore, 06-1398); anti-β-tubulin conjugated to Alexa Fluor 555 (Cell Signaling Technology, 2116); anti-γ-tubulin (Sigma, T-3559 (1:3,000 for WB and 1:3,00 for IF)); anti-Kin-2 (Origene, TA500505 (1:2,000 for WB)); anti-β-integrin (BD Pharmingen, 9EG7 (1:75 for FACS)); anti-phospho (Y-416 Src (Cell Signaling Technology, 2101); anti-Paxillin (BD Transduction Laboratories, 610052 (1:300 for IF)); anti-Vinculin (Sigma, V-4139). All antibodies were used at 1:1,000 for WB and 1:200 for IF unless otherwise stated. Clonogenic assays Cells were transfected and immediately plated at low density. Upon appearance of colonies, 10–14 days after transfection, cells were washed in ice cold PBS (two times) and fixed in methanol (−20 °C cooled) on ice for 10 min. Colonies were stained with crystal violet solution (0.5% crystal violet (w/v) in 25% methanol (v/v)) for 10 min at room temperature. Plates were washed five times in water and allowed to dry and number of colonies counted. How to cite this article: Patel, H. et al. Kindlin-1 regulates mitotic spindle formation by interacting with integrins and Plk-1. Nat. Commun. 4:2056 doi: 10.1038/ncomms3056 (2013).